Genome-wide association study identifies novel genetic variants contributing to variation in blood metabolite levels Metabolites are small molecules involved in cellular metabolism, which can be detected in biological samples using metabolomic techniques. Here we present the results of genome-wide association and meta-analyses for variation in the blood serum levels of 129 metabolites as measured by the Biocrates metabolomic platform. In a discovery sample of 7,478 individuals of European descent, we find 4,068 genome- and metabolome-wide significant ( Z -test, P <1.09 × 10 −9 ) associations between single-nucleotide polymorphisms (SNPs) and metabolites, involving 59 independent SNPs and 85 metabolites. Five of the fifty-nine independent SNPs are new for serum metabolite levels, and were followed-up for replication in an independent sample ( N =1,182). The novel SNPs are located in or near genes encoding metabolite transporter proteins or enzymes ( SLC22A16 , ARG1 , AGPS and ACSL1 ) that have demonstrated biomedical or pharmaceutical importance. The further characterization of genetic influences on metabolic phenotypes is important for progress in biological and medical research. Metabolite levels in human blood reflect the physiological state of the body, and may differ between individuals because of variation in genetic makeup and environmental exposure [1] . The study of the genetic contribution to variation in metabolite levels is an important basis for improved aetiological understanding, prevention, diagnosis and treatment of complex disorders [1] , [2] . Modern high-throughput metabolomics enables the cost-effective measurement of large metabolite panels in blood samples obtained from many individuals. The data generated by such metabolomic experiments have been combined with genotypic data in several recent genome-wide association (GWA) studies [2] , [3] , [4] , [5] , [6] , [7] , [8] , [9] , [10] , [11] , [12] . Indeed, the combined investigation of large numbers of genetic variants and large numbers of metabolic traits is beginning to draw a systems-wide overview of genetic influences on human metabolism [11] . However, the heritability estimates from twin and family studies [9] , [10] , [11] , [13] suggest that additional genetic variants influencing variation in serum metabolite levels remain to be found in GWA studies. In the current study, we set out to further characterize the genetic contribution to variation in human blood metabolite levels. We perform GWA and meta-analyses for the concentrations of 129 serum metabolites in seven independent cohorts, with replication analyses in one additional cohort. To functionally characterize the significant single-nucleotide polymorphism (SNP)-metabolite associations, we integrate the results of the GWA meta-analyses with those from gene expression analysis in whole blood and the liver. Finally, we compare the variance explained by significantly associated SNPs with heritability estimates for each metabolite. We identify 4,068 significant SNP-metabolite associations, involving 59 independent SNPs and 85 different metabolites. Five of the fifty-nine independent SNPs are novel for serum metabolite levels. The newly found SNP-metabolite associations may lead to a better understanding of cardiovascular and metabolic disease, and may have implications for chemotherapy. Our findings contribute to the understanding of human metabolism. Discovery meta-analysis of GWA scans Primary genetic association analyses were carried out in seven cohorts (TwinsUK, KORA, EGCUT, LLS, QIMR, ERF and NTR) with a combined sample size of 7,478 individuals. 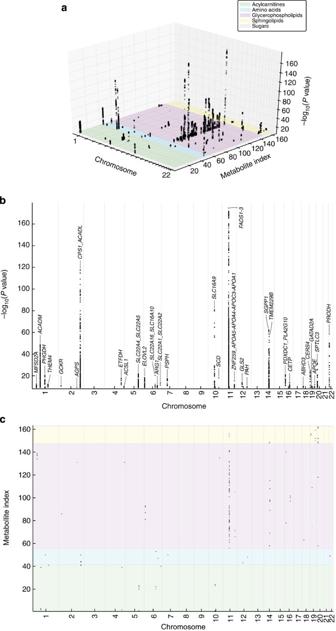Figure 1: Manhattan plots for all metabolites targeted by the Biocrates AbsoluteIDQ p150 kit (N=[1,497, 7,478]). These plots graphically display thePvalues for significant (Z-testP<1.09 × 10−9) SNP-metabolite associations in the discovery phase in the current study. (a) A three-dimensional view; orthogonal projections are given in (b) and (c). SNPs are arranged according to genomic location along the ‘Chromosome’ axes. The ordering of the metabolites along the ‘Metabolite index’ axes is equal in bothaandc, and equal to that inSupplementary Table 3. Inaandb, all data points are displayed semi-transparent and therefore opaque regions in the plot indicate clusters of significant associations. Inb, loci are identified by most plausible causal gene or, if no plausible genes found, by nearest gene. Where multiple plausible genes could be identified at the locus (possibly for different metabolites), the gene names are separated by an underscore (‘_’) in the locus name. Inc, the size of the markers scales linearly with -log10(Pvalue). This Figure is also supplied as a movie (seeSupplementary Movie 1). Characteristics of the study participants included in the analyses (all of European descent) are given in Supplementary Table 1 . 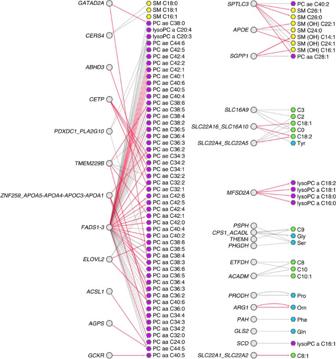Figure 2: Associations between loci and metabolites detected in stage 1 meta-analysis in the current study (N=[1,588, 7,478]). Loci significantly associated with at least one metabolite are depicted as grey circles. Biochemical classes (seeSupplementary Table 3) of the metabolites (hexagons) are indicated by node colours: green, acylcarnitines; blue, amino acids; purple, glycerophospholipids; yellow, sphingolipids. Arrows point from each locus to the associated metabolite(s); arrow widths scale linearly with -log10(associationPvalue). Grey arrows denote previously known associations; red arrows denote associations that were newly discovered on the basis of stage 1 meta-analysis in the current study (that is, either associations with new SNPs for serum metabolite levels, or an association of a known SNP with a new metabolite with respect to 11 previous GWA studies for serum metabolite levels2,3,4,5,6,7,8,9,10,11,12). Loci are identified by most plausible causal gene or, if no plausible genes found, by nearest gene. Where multiple plausible genes could be identified at the locus (possibly for different metabolites), the gene names are separated by an underscore (‘_’) in the locus name. At this significance threshold (P=1.09 × 10−9), the locus-metabolite association network separates into 12 connected components or disconnected sub-networks, each including metabolites from maximally two chemical classes. This figure was created using Cytoscape52. Within each cohort, SNP genotypes were imputed and analysed for association with the concentrations of each metabolite, assuming a linear model of association and correcting for population stratification (see Methods and Supplementary Table 2 ). Supplementary Tables 3–5 and Supplementary Data 1 list the characteristics of the 129 metabolites (18 acylcarnitines, 14 amino acids, 82 glycerophospholipids, 14 sphingolipids and hexose) that were measured in the serum samples from all study participants using the Biocrates platform. The cohort-level GWA results were pooled in inverse variance-weighted, fixed-effects meta-analysis. The values of the genomic control lambda (λ GC , applied to the individual cohort-level results for each metabolite before meta-analysis) varied between 0.976 and 1.081 across all metabolites and cohorts (see Supplementary Table 6 ), suggesting little residual influence on the GWA results of population stratification and other potential confounders. A three-dimensional Manhattan plot providing an overview of the association P values in the discovery phase for all metabolites is given in Fig. 1 ; two-dimensional Manhattan plots and quantile-quantile plots for each metabolite separately are given in Supplementary Figs 1 and 2 , respectively. Overall, 4,068 SNP-metabolite associations reached genome- and metabolome-wide significance ( Z -test, P <1.09 × 10 −9 ), which reduced to 123 associations involving 59 independent SNPs and 85 different metabolites. Of these 123 associations (listed in Supplementary Data 2 ), 4 represented secondary association signals according to approximate conditional analysis. Regional association plots, showing the association signals in the regions surrounding the lead metabolomic SNPs, are given for all 123 associations in Supplementary Fig. 3 . SNPs representing independent association signals were aggregated into 31 genomic loci, which are listed in Supplementary Data 3 . Figure 2 depicts all associations between loci and metabolites as detected in the discovery phase. Figure 1: Manhattan plots for all metabolites targeted by the Biocrates AbsoluteIDQ p150 kit ( N =[1,497, 7,478]). These plots graphically display the P values for significant ( Z- test P <1.09 × 10 −9 ) SNP-metabolite associations in the discovery phase in the current study. ( a ) A three-dimensional view; orthogonal projections are given in ( b ) and ( c ). SNPs are arranged according to genomic location along the ‘Chromosome’ axes. 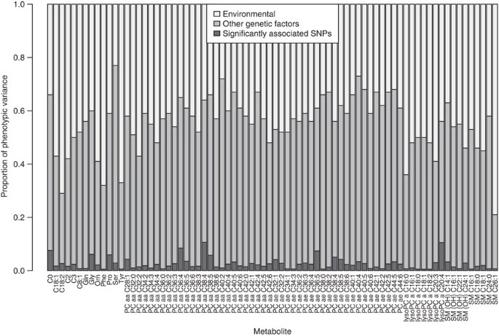Figure 3: Decomposition of variation in serum metabolite levels. This figure displays the proportions of variance in serum metabolite level explained by significantly associated SNPs; heritability not explained by significantly associated SNPs and unexplained (environmental) variance. Seventy-six metabolites are included for which both heritability estimates (monozygotic twin correlations taken from reference13;N=181 pairs; Pearson correlation) were available, and that displayed genome- and metabolome-wide associations with SNPs in stage 1 GWA meta-analysis in the current study (N=[1,588, 7,478]). Proportion of variance explained by significantly associated SNPs was estimated as Pearson’s phi coefficient squared. Metabolites are grouped according to biochemical class. The ordering of the metabolites along the ‘Metabolite index’ axes is equal in both a and c , and equal to that in Supplementary Table 3 . In a and b , all data points are displayed semi-transparent and therefore opaque regions in the plot indicate clusters of significant associations. In b , loci are identified by most plausible causal gene or, if no plausible genes found, by nearest gene. Where multiple plausible genes could be identified at the locus (possibly for different metabolites), the gene names are separated by an underscore (‘_’) in the locus name. In c , the size of the markers scales linearly with -log 10 ( P value). This Figure is also supplied as a movie (see Supplementary Movie 1 ). Full size image Figure 2: Associations between loci and metabolites detected in stage 1 meta-analysis in the current study ( N =[1,588, 7,478]). Loci significantly associated with at least one metabolite are depicted as grey circles. Biochemical classes (see Supplementary Table 3 ) of the metabolites (hexagons) are indicated by node colours: green, acylcarnitines; blue, amino acids; purple, glycerophospholipids; yellow, sphingolipids. Arrows point from each locus to the associated metabolite(s); arrow widths scale linearly with -log 10 (association P value). Grey arrows denote previously known associations; red arrows denote associations that were newly discovered on the basis of stage 1 meta-analysis in the current study (that is, either associations with new SNPs for serum metabolite levels, or an association of a known SNP with a new metabolite with respect to 11 previous GWA studies for serum metabolite levels [2] , [3] , [4] , [5] , [6] , [7] , [8] , [9] , [10] , [11] , [12] ). Loci are identified by most plausible causal gene or, if no plausible genes found, by nearest gene. Where multiple plausible genes could be identified at the locus (possibly for different metabolites), the gene names are separated by an underscore (‘_’) in the locus name. At this significance threshold ( P =1.09 × 10 −9 ), the locus-metabolite association network separates into 12 connected components or disconnected sub-networks, each including metabolites from maximally two chemical classes. This figure was created using Cytoscape [52] . Full size image Five independent SNPs had not been associated with variation in serum metabolite levels in previous GWA studies (see Table 1 ). To further interpret the association of the remaining 54 SNPs with serum metabolite concentrations, we compared our findings with those from 11 published GWA studies [2] , [3] , [4] , [5] , [6] , [7] , [8] , [9] , [10] , [11] , [12] for which at least one of the included metabolites overlapped with the current study. The identified associations of known SNPs with metabolites that were significant in discovery stage meta-analysis in the current study and that had not been reported in those previous studies are highlighted in Fig. 2 and in Supplementary Data 2 . Table 1 Novel SNPs for serum metabolite levels identified in the current study. Full size table Replication analysis Replication analyses were performed in an independent sample ( N =1,182) from the KORA S4 cohort (hereafter KORA S4 replication sample) for the five new SNPs for serum metabolite levels that had been found in the discovery phase meta-analysis. The associations with their most strongly associated metabolite were replicated for four of these five novel SNPs; the only non-replicated association was that between SNP rs7582179 and metabolite PC ae C44:5. Although the effect sign was concordant between the discovery set and the KORA S4 replication sample ( Table 1 ), this association was significant in the discovery phase for the NTR and KORA cohorts only (see Supplementary Fig. 4 ). Integration with gene expression analysis results We integrated the results of the metabolomics discovery stage GWA meta-analysis with the results of gene expression analyses in whole blood and the liver. In whole blood, both cis and trans expression quantitative trait locus ( cis- eQTL and trans -eQTL, respectively) analyses were performed in two different samples originating from the United Kingdom, the Netherlands and Estonia: the Dutch NTR-NESDA sample ( N =5,071) and the Fehrmann-EGCUT sample comprising data from three cohorts that were meta-analysed (total N =2,360; see Methods and Supplementary Methods ). The results of cis -eQTL analysis for lead metabolomic SNPs showing overlap with cis -eQTL SNPs are given for the NTR-NESDA and Fehrmann-EGCUT samples in Supplementary Data 4 and 5 , respectively. Significant (false discovery rate<0.05) trans -eQTL effects for lead metabolomic SNPs in the Fehrmann-EGCUT sample are listed in Supplementary Data 6 . We did not detect trans -eQTL effects for the lead metabolomic SNPs in the NTR-NESDA sample. Thirty-five lead metabolomic SNPs identified cis -eQTLs in at least one of the searched tissues (i.e., whole blood and/or the liver) with a ( t -, Z - or Kruskal-Wallis test) P <0.001, defining a total of 67 SNP-gene pairs and 28 different genes (see Supplementary Data 7 ). The cis -eQTL analysis results were used to support the annotation of likely causal genes to loci that displayed significant association with variation in serum metabolite concentrations in the discovery stage meta-analysis (see Supplementary Data 3 ). Of the 28 genes, 14 were predicted to be causal on the basis of our annotation and the other 14 were predicted to be non-causal. Variance explained It has been described previously that a relatively small number of genetic variants can explain a relatively large proportion of the variance observed for serum metabolite levels [4] , [5] , [9] . Therefore, we compared the variance in serum metabolite levels explained by significantly associated SNPs, with the heritability as estimated in a monozygotic twin sample from the NTR cohort ( N =181 pairs; see Fig. 3 ) [13] . Among all metabolites, the largest proportion of phenotypic variance was explained for C9 (13%; see Supplementary Data 2 ). In the current study, this metabolite associated significantly with SNPs in the THEM4 and CPS1_ACADL loci. The largest proportion of heritability was explained for lysoPC a C20:4 (19%; corresponding with 10% of the phenotypic variance), which was associated with a SNP in the FADS1–3 locus. The results of polygenic score (PGS) analyses (see Supplementary Fig. 5 and Supplementary Note 1 ) suggest different genetic background of variation in serum levels for different metabolites, ranging from close-to-monogenic to highly polygenic. Figure 3: Decomposition of variation in serum metabolite levels. This figure displays the proportions of variance in serum metabolite level explained by significantly associated SNPs; heritability not explained by significantly associated SNPs and unexplained (environmental) variance. Seventy-six metabolites are included for which both heritability estimates (monozygotic twin correlations taken from reference [13] ; N =181 pairs; Pearson correlation) were available, and that displayed genome- and metabolome-wide associations with SNPs in stage 1 GWA meta-analysis in the current study ( N =[1,588, 7,478]). Proportion of variance explained by significantly associated SNPs was estimated as Pearson’s phi coefficient squared. Metabolites are grouped according to biochemical class. Full size image We set out to enhance the current understanding of the genetic underpinnings of variation in circulating metabolite levels in humans. To this end, we employed a well-established targeted metabolomics platform (Biocrates) in combination with genome-wide SNP genotyping and imputation in eight independent cohorts of European descent. By meta-analysis of GWA analyses carried out for each of 129 metabolites measured in the serum samples of all individual study participants, the current study identified 123 significant SNP-metabolite associations between 59 independent SNPs and 85 different metabolites. Five of the independent SNPs were new for variation in serum metabolite levels. Consistent with previous reports, for the majority of all 59 independent SNPs we were able to annotate a likely causal gene, which in most cases encoded a metabolite transporter protein or enzyme. The five new SNPs for serum metabolite levels are also all located nearby such genes, and their associations with metabolites tend to match the known function of these genes. SNP rs7582179 in the AGPS gene is associated with the choline plasmalogen PC ae C44:5. Mutations in AGPS (encoding the enzyme alkylglycerone phosphate synthase) are known to cause rhizomelic chondrodysplasia punctata type 3 (RCDP3; OMIM:600121 (ref. 14 )), a rare autosomal recessive disorder that is fatal, with death occurring often early in childhood. Clinically, RCDP3 is characterized by significantly delayed and abnormal physical and mental development, with shortness of the proximal limb bones (‘rhizomelia’) being one of the hallmarks. RCDP3 has been shown to result from reduced production of plasmalogens (a type of ether phospholipids) by alkylglycerone phosphate synthase in peroxisomes. The association in the current study of a SNP within the AGPS gene with the serum concentration of the choline plasmalogen PC ae C44:5 is therefore perfectly concordant with the known gene-disease link between AGPS and RCDP3. PC ae C44:5 also associated significantly with the new SNP rs7700133 located near the ACSL1 gene, encoding long-chain acyl CoA synthetase 1. Previous studies have shown links between genetic and transcriptional variation of ACSL1 and the metabolic syndrome [15] , [16] . The new SNP rs12210538, located within the SLC22A16 gene, associated with the two acylcarnitines C18:1 and C18:2. This gene encodes a carnitine transporter that mediates the uptake of anticancer drugs such as bleomycin and doxorubicin into tumour cells, and its activity correlates with treatment response [17] , [18] . Significant associations were found for two SNPs (rs17657817 and rs2246012) located inside the ARG1 gene (coding for the enzyme arginase) with serum concentrations of the amino acid ornithine that participates in the urea cycle. Importantly, the global arginine bioavailability ratio (that is, the ratio of arginine to ornithine and citrulline [19] ) is of interest as a potential biomarker for endothelial dysfunction, which is a known risk factor for the development of cardiovascular disease [20] . The two newly identified SNPs associated with serum ornithine levels might now be used as instrumental variables in cost-effective Mendelian randomization studies in large samples of individuals, to investigate the possible causal relationship among ornithine, endothelial dysfunction and subsequent cardiovascular disease [21] . Among three meta-analyses of coronary artery disease and myocardial infarction as carried out by the CARDIoGRAMplusC4D Consortium, the association with SNP rs2246012 was the strongest in the CARDIoGRAM GWA study ( P =0.002) involving 22,233 cases and 64,762 controls [22] . This suggests that the link between genetic variation at SNP rs2246012 and variation in serum ornithine levels as identified in the current study will indeed be useful to further establish the possible link between the ARG1 gene and cardiovascular disease. We compared the significant SNP-metabolite associations from the current study with those reported in 11 previous publications that employed high-resolution methods to assay the serum metabolome. For several SNPs that were associated with variation in metabolite levels in the previous studies, we identified new associations with individual metabolites. These new associations strengthen the evidence for the associations of these known SNPs with specific metabolites, demonstrating their extended effect on phenotypes that are closely related to the metabolites with which their association was discovered initially [4] , [23] . Also, it has been demonstrated that GWA studies with the more refined metabolic phenotypes provided by metabolomics often yield effect sizes that are larger than those observed in GWA studies of composite measures such as high-density lipoprotein cholesterol, suggesting that these more refined metabolomic phenotypes provide better intermediate traits [8] , [9] . In this context, it is interesting to note that the large proportion of explained heritability we observed for lysoPC a C20:4 (19%) was caused exclusively by the association with a single SNP in the FADS1–3 locus, an observation that is in line with the results from previous studies [4] , [5] , [9] . In conclusion, the results obtained in the current study contribute to the understanding of the genetic background of variation in serum metabolite levels, and are important for further progress in biomedical and pharmaceutical research. Participants The meta-analysis included GWA data from 7,478 participants from seven cohorts originating from five countries (the Netherlands, Germany, Australia, Estonia and the United Kingdom). The independent test sample (‘KORA S4 replication sample’) consisted of 1,182 additional KORA participants. The following local research ethics committees approved the individual studies: KORA, Ethics Committee of the Bavarian Medical Association (Bayerische Landes-ärztekammer); NTR, Central Ethics Committee on Research Involving Human Subjects of the VU University Medical Center, Amsterdam; EGCUT, Ethics Review Committee on Human Research of the University of Tartu; TwinsUK, St Thomas’ Hospital ethics committee; ERF, medical ethics board of the Erasmus MC Rotterdam, the Netherlands; LLS, Medical Ethical Committee of the Leiden University Medical Centre; QIMR, QIMR Human Research Ethics Committee. Informed consent was obtained from all participants. Sample characteristics for all cohorts included in this study and detailed study sample descriptions are given in Supplementary Table 1 and in the Supplementary Methods , respectively. Biocrates metabolite quantification Targeted metabolomic measurements were performed using electrospray–flow injection analysis–tandem mass spectrometry methods and the Biocrates AbsoluteIDQ p150 kit (BIOCRATES Life Sciences AG), which enables quantification of a total of 163 metabolites (see Supplementary Table 3 for an overview of all metabolites targeted by this kit) [24] . The method of AbsoluteIDQ p150 kit has been proven to be in conformance with FDA Guideline ‘Guidance for Industry—Bioanalytical Method Validation (May 2001)’ [25] , which implies proof of reproducibility within a given error range. For all cohorts, metabolite measurements were carried out at the Metabolomics Platform of the Genome Analysis Center at the Helmholtz Zentrum München, Germany as per the manufacturer’s instructions [4] , [24] , [26] , [27] . In brief, the used metabolomic measurement technique is based on a targeted profiling scheme that is used to quantitatively screen for known small-molecule metabolites by multiple reaction monitoring, neutral loss and precursor-ion scans. Internal standards served as reference for the calculation of all metabolite concentrations, which are reported as micromolar. Data evaluation for quantification of metabolite concentrations and quality assessment have been performed with the MetIDQ software package, which is an integral part of the AbsoluteIDQ kit. Stability of the assay was assessed using the measurement results of five aliquots of the same reference blood sample on every plate. Quality control of the Biocrates metabolite concentration measurement data was performed by each participating cohort as follows [27] : for each cohort, metabolite profile measurements for all individuals were performed on multiple plates. For each metabolite i and plate j , the coefficient of variation (CV i,j ) was calculated as: , where the standard deviation (s.d.) and mean were calculated over all reference measurements per plate j (five per plate). Summary statistics for the metabolite concentration data for each cohort were compared with the measurement detection limit specifications as reported by the manufacturer of the AbsoluteIDQ p150 kit (BIOCRATES). A metabolite was excluded from further analyses for a particular cohort if its concentration measurement data did not meet all of the following criteria: (i) mean CV i over all plates <25%; (ii) ≤5% missing values; (iii) median >lower limit of quantification (for metabolites reported as absolute concentrations) or >limit of detection (for semiquantitatively measured metabolites). Outlying metabolite concentration values (data points) and outlying samples were also removed, and the missing data points were imputed with the ‘R’ [28] package ‘mice’ [27] . The resulting concentration data for each metabolite were natural log-transformed in order to attain a normal distribution. Throughout the article, names of lipids detected by the Biocrates AbsoluteIDQ p150 platform are abbreviated as follows: acylcarnitines, C x:y ; hydroxylacylcarnitines, C(OH) x:y ; dicarboxylacylcarnitines, C x:y -DC; sphingomyelins, SM x:y ; N -hydroxylacyloylsphingosylphosphocholine, SM (OH) x:y ; phosphatidylcholines, PC (aa=diacyl, ae=acyl-alkyl). Lipid side chain composition is abbreviated as C x:y , where x denotes the number of carbons in the side chain and y the number of double bonds. Association analyses and meta-analyses Genome-wide SNP genotyping was performed in each cohort with standard genotyping technologies (see Supplementary Table 2 and Supplementary Methods ). For the samples contributing to the stage 1 (discovery) meta-analysis, imputation was conducted with reference to HapMap phase 2 build 36 release 22 or 24 CEU (Utah residents of Northern and Western European ancestry) [29] phased genotypes. For the KORA S4 replication sample, SNP genotypes were imputed against the 1,000 g phase1 integrated haplotypes reference set. Association analysis was performed assuming a linear regression model for each SNP, adjusting for relatedness, age, sex and study specific (for example, ancestry-informative principal component scores) covariates as necessary (see Supplementary Table 2 ). Positions of all SNPs described in the current manuscript were mapped to those as in the HapMap 2 Build 36 release 24 reference set (hg18). Meta-analysis of GWA results obtained in the cohorts participating in stage 1 was performed as follows: the expected minor allele count (eMAC) was computed at the cohort level for each SNP as where N is the study sample size, MAF is the minor allele frequency and I A is the SNP genotype imputation quality measure. SNPs for which eMAC<25 were filtered out of the GWA results for the cohort under consideration. After applying genomic control at the individual cohort level, two independent analysts carried out additive model fixed-effects meta-analysis of association data for imputed autosomal SNPs, using two different software packages (METAL [30] and GWAMA [31] ). For a given SNP, cohort-specific effect size estimates were weighted inversely with their variance. Throughout the manuscript, we report the P values as resulting from Z -tests of association as carried out by METAL. A P value equal to 5.0 × 10 −8 was adopted as the threshold for genome-wide suggestive association between a SNP and the concentration of a metabolite, based on the approximate number of independent SNPs in samples of European ancestry [32] . To obtain a threshold for significant association, taking account of the number of metabolites tested and their intercorrelations, the threshold value for suggestive association was divided by the number of independent tests (Meffli) in the metabolomic data as estimated using the method of Li and Ji [33] . The value of Meffli was estimated on the basis of the metabolite profiling data in two independent cohorts (ERF and NTR). Meffli was estimated to be equal to 46 in both ERF and NTR, rendering the P value threshold for genome- and metabolome-wide significance in the present study to be equal to 5.0 × 10 −8 /46=1.09 × 10 −9 . Definition of loci and secondary signals analysis Independent signals of association were identified in the GWA meta-analysis results for each metabolite separately, using the linkage disequilibrium-based ‘clumping’ procedure as implemented in PLINK [34] . This procedure takes all SNPs that show a P value of association with a phenotype below a threshold (‘—clump-p1’), and forms clumps of these ‘index’ SNPs together with all other SNPs that are in linkage disequilibrium with (controlled by the parameter ‘—clump-r2’) and in physical proximity (controlled by parameter ‘—clump-kb’) to these index SNPs. For the current study, we used the following parameter settings: ‘—clump-p1’, 5.0 × 10 −8 ; ‘—clump-r2’, 0.1; ‘—clump-kb’, 1,000. As input for the ‘clumping’ procedure, we used association P values from the discovery phase meta-analysis results and linkage disequilibrium patterns as estimated from the HapMap 2 Build 36 release 24 reference set. For each metabolite separately, secondary association signals at a locus were verified by approximate conditional analysis as implemented in GCTA [35] . In this analysis, the association for the secondary association signal ‘top’ SNP (that is, the SNP with the lowest P value of association with variation in serum metabolite level at the secondary association signal) was conditioned on the top SNP for the locus and metabolite under consideration. As input for the approximate conditional analysis, we used the discovery phase GWA meta-analysis results and the imputed SNP genotype data from the NTR cohort as a reference for LD structure [36] . We report only secondary signal top SNPs for which the P value remained <1.09 × 10 −9 in this approximate conditional analysis. In the current manuscript, the term ‘lead metabolomic SNP’ refers to a top SNP at a locus or secondary association signal for one or more metabolites. We identified genomic loci significantly associating with metabolite levels by grouping lead metabolomic SNPs located within 1 Mb from each other over all metabolites. Identification of new SNP–metabolite associations The approach used in the current study to identify novel associations between SNPs and serum metabolite levels is described in Supplementary Fig. 6 and in the Supplementary Methods . In brief, we applied two complementary methods: the first method identified novel SNPs associated with variation in serum metabolite levels, and the second method identified novel SNP-metabolite associations with respect to 11 previous GWA studies that included at least one metabolite that was also included in the current study. Replication analyses Replication analyses were performed in the KORA S4 replication sample for the associations of the five new SNPs for serum metabolite levels (listed in Table 1 ) with their lead metabolites (that is, the metabolites that were most strongly associated with these SNPs in the discovery phase meta-analysis). Lookup of association with cardiovascular disease Data on coronary artery disease/myocardial infarction have been contributed by CARDIoGRAMplusC4D investigators and have been downloaded from www.CARDIOGRAMPLUSC4D.ORG . We performed a lookup of the associations with SNP rs2246012 in the results from all three meta-analyses as provided on this website [22] , [37] , [38] . Association and Manhattan plots For each lead metabolomic SNP, the LocusZoom [39] tool was used to generate association plots in the region between 500 kb before the locus minimum position and 500 kb after the locus maximum position. Manhattan plots for each metabolite were generated based on the discovery phase meta-analysis results using in-house developed Python [40] code. SNP annotation To facilitate the manual process of selecting plausible candidate genes for each locus, we used an automated workflow developed in-house to generate reports containing the associated protein, enzyme, metabolic reaction, pathway and disease phenotypes of each gene within a ±500 kb window of each lead metabolomic SNP. SNPs within this window that were published in GWAS Catalog [41] or in GTEx-eQTL ( http://www.ncbi.nlm.nih.gov/gtex/GTEX2 ) were also listed. In detail, the reports created by our workflow were based on the NCBI-Gene ( http://www.ncbi.nlm.nih.gov/gene ), GTEx-eQTL, GWAS Catalog, ConsensusPathDB [42] , UniProtKB [43] , OMIM [44] , Gene Ontology [45] , TCDB [46] , ExPASy [47] and KEGG databases [48] . These databases had been downloaded earlier from the respective File Transfer Protocol servers and have been integrated offline in MATLAB (R2009a, The Mathworks Inc.). Overlap of lead metabolomic SNPs with cis -eQTL SNPs was also used as evidence to support the annotation of likely causal genes to loci. In case no biologically plausible gene could be found, the locus was given the name of the nearest gene; a similar approach was followed in the study by Shin et al . [11] Variance explained We estimated the proportion of phenotypic variance explained by each independent association signal (lead SNP for a locus or secondary association signal) as Pearson’s phi coefficient squared: where ; N is the sample size in the discovery phase meta-analysis for the SNP–metabolite association under consideration; is the ordinary least-squares estimate of (that is, the regression coefficient for the SNP as estimated in the discovery phase meta-analysis); and is its standard error. For each metabolite, we added up the proportions of variance in metabolite level explained by independent association signals to estimate the total proportion of phenotypic variance explained. We also estimated for each metabolite the proportion of heritability of metabolite level variability explained by approximately independent association signals. As an estimate of heritability for this analysis we used the monozygotic twin correlations for each metabolite, based on data from 181 pairs from the NTR cohort [13] . The proportion of heritability in metabolite level variation explained by independent association signals was estimated by dividing the proportion of phenotypic variance explained by independent association signals, by the monozygotic twin correlation. The total proportion of heritability explained for a particular metabolite was estimated by adding up the proportions of variance explained by all approximately independent association signals for that metabolite. PGS analysis We investigated evidence for the polygenic nature of variation in serum metabolite levels by building a multi-SNP predictor from the meta-analysis results for each metabolite to predict the levels of the same metabolite in an independent target cohort (KORA S4 replication sample). Such a multi-SNP predictor, or PGS, reflects the weighted sum of multiple SNPs associated with a phenotype. The discovery meta-analysis forms the basis to select SNPs based on liberal significance thresholds (for example, 0.001, 0.01 and so on). In the target sample, PGSs are calculated for each individual for each set of SNPs by multiplying the number of effect alleles per SNP (0, 1 or 2) with the beta from the meta-analysis, summed over all SNPs in the set of SNPs. We performed the PGS analysis [49] using the regression coefficients (betas) from the discovery phase meta-analyses as weights. Analyses were performed for the 127 metabolites for which concentration data were available both in the discovery sample and in the KORA S4 target sample. For each of these metabolites, SNPs representing approximately independent association signals were selected in the discovery phase meta-analysis results using the PLINK clumping procedure. SNPs with P values of association with metabolite concentration levels in the discovery meta-analysis below the following thresholds were included: P <1.0 × 10 −8 ; P <1.0 × 10 −7 ; P <1.0 × 10 −6 ; P <1.0 × 10 −5 ; P <1.0 × 10 −4 ; P <1.0 × 10 −3 ; P <1.0 × 10 −2 ; P <5.0 × 10 −2 ; P <0.1; P <0.2; P <0.3; P <0.4; P <0.5; P <0.6; P <0.7; P <0.8; P <0.9; P <1.0. For each clump of SNPs, the index SNP was taken for possible inclusion in the score computation. From the resulting set of SNPs eligible for inclusion in the PGS analysis, A/T and G/C SNPs for which (0.35<MAF<0.50) were excluded because these SNPs are potentially ambiguous and therefore may lead to spurious association in the case of strand flips [50] . From the imputed SNP genotype data for the KORA S4 target sample, the SNPs corresponding with the remaining clump index SNPs were selected. A PGS was constructed for each individual in the KORA S4 replication sample using the ‘—score’ procedure as implemented in PLINK v. 1.07 ( http://pngu.mgh.harvard.edu/~purcell/plink/profile.shtml) . The resulting PGS was included as a covariate in a multiple linear regression analysis that was similar to the regression that was carried out in the primary single SNP-based GWA analysis: where y represents log(metabolite) values, and the study-specific covariates include adjustments for, for example, population stratification (and thus β 4 can be a vector). The Biocrates metabolite values were obtained and preprocessed using the same methods as described for the primary GWA in the Section ‘Biocrates metabolite quantification’. The proportion of variance explained by the PGSs was assessed by comparing the raw (that is, unadjusted) R 2 values for the ‘full’ model (that is, a model including the genetic score as a covariate) with the raw R 2 values when fitting a ‘reduced’ model that did not include the genetic score as a covariate [51] . The significance of the association of the PGSs with serum metabolite levels was estimated on the basis of the P value of association for β 1 according to the full model. EQTL analyses Data from two independent samples originating from the United Kingdom, the Netherlands and Estonia (the Dutch NTR-NESDA sample and the Fehrmann-EGCUT sample) were used for cis - and trans -eQTL mapping in whole blood. Details of these analyses, and of the integration of the cis -eQTL analysis results with the results from the metabolomics genome-wide meta-analysis, are provided in the Supplementary Methods . We also assessed the overlap of lead metabolomic SNPs with cis -eQTL signals in the liver as catalogued in the GTEx-eQTL database, following the method of Shin et al . [11] : for each lead metabolomic SNP, we retrieved all SNPs with r 2 >0.8 in the 1000 Genomes Project pilot phase (CEU population). All cis -eQTLs within a 1-Mb window centred on the lead SNP were retrieved from the GTEx-eQTL database, and the best eQTL P value was noted. The cis -eQTL results for which overlap with lead metabolomic SNPs was shown and that displayed association P values <0.001 are given in Supplementary Data 7 . Meta-analysis The full meta-analysis results for all metabolites are available at www.tweelingenregister.org/engagebiocratesgwama Accession codes. The metabolomic data described in this manuscript are uploaded to MetaboLights and are available under the accession code MTBLS192. How to cite this article: Draisma, H.H.M. et al . Genome-wide association study identifies novel genetic variants contributing to variation in blood metabolite levels. Nat. Commun . 6:7208 doi: 10.1038/ncomms8208 (2015).